Reversible cyclic deformation mechanism of gold nanowires by twinning–detwinning transition evidenced fromin situTEM Mechanical response of metal nanowires has recently attracted a lot of interest due to their ultra-high strengths and unique deformation behaviours. Atomistic simulations have predicted that face-centered cubic metal nanowires deform in different modes depending on the orientation between wire axis and loading direction. Here we report, by combination of in situ transmission electron microscopy and molecular dynamic simulation, the conditions under which particular deformation mechanisms take place during the uniaxial loading of [110]-oriented Au nanowires. Furthermore, by performing cyclic uniaxial loading, we show reversible plastic deformation by twinning and consecutive detwinning in tension and compression, respectively. Molecular dynamics simulations rationalize the observed behaviours in terms of the orientation-dependent resolved shear stress on the leading and trailing partial dislocations, their potential nucleation sites and energy barriers. This reversible twinning–detwinning process accommodates large strains that can be beneficially utilized in applications requiring high ductility in addition to ultra-high strength. The plastic deformation of dislocation-free metal nanowires is known to initiate at a stress level on the order of the theoretical strength [1] , [2] , [3] , [4] , [5] . In the absence of preexisting dislocations, the onset of plastic deformation relies on the nucleation of dislocations, which usually requires a much higher stress than that needed to operate dislocation sources present in the bulk material. Moreover, upon nucleation, dislocations glide swiftly to the nanowire surface with a very limited chance of interaction or multiplication [6] , [7] . Therefore, the plastic flow of nanowires requires continued activation of dislocation nucleation processes. Depending on the nature of the nucleation mechanism, diverse mechanical responses may result during plastic deformation. Shrinking the size of metallic structures not only leads to an increase of strength (that is, the ‘smaller is stronger’ size effect [8] ), but also to a change in the deformation mechanism [9] , [10] , [11] , [12] , [13] , [14] . For face-centered cubic (fcc) metals, a transition from dislocation slip to deformation twinning has been reported when their characteristic size (for example, grain size, film thickness, wire or pillar diameter) decreased below several 10 nm [9] , [10] , [11] , [12] . In the case of uniaxial deformation of fcc metal nanowires, the deformation mechanism can also change with the loading condition. According to recent molecular dynamics (MD) simulations, ultra-thin Au [110] nanowires (diameters of a few nm) deform predominantly by dislocation slip in compression, but in tension by deformation twinning [13] . Conversely, under the same loading conditions, the deformation mechanism also changes with the axial orientation of nanowire [13] , [14] . Deformation twinning and dislocation slip occur through dislocation processes operating on the same set of slip systems, so they are in direct competition. In the absence of preexisting dislocations or twins, however, the first step in both slip and twinning is the nucleation of a leading partial dislocation. The critical step determining the deformation mechanism is whether the leading partial dislocation is subsequently followed by the nucleation of a trailing partial dislocation on the same slip plane, thereby forming a perfect dislocation, the nucleation of another leading partial dislocation on a separate slip plane, thus leading to partial slip, or on an adjacent slip plane, resulting in the formation of a two-layer embryonic twin, in other words, an extrinsic stacking fault. In the case of uniaxial deformation of nanowires, the differences in the work done by the resolved shear stress on each pair of partial dislocations required for slip and twinning processes should be the primary criterion in determining the deformation mode at a specific loading condition [15] . Detwinning should be considered as an alternative deformation mode when twins are present in the tested nanowires. Detwinning has been observed experimentally during the deformation of nano-twinned grains [16] and near the crack tip in twinned fcc metals [17] . MD simulations have predicted that Ni [110] nanowires with a diameter smaller than 2 nm exhibit shape memory and pseudoelastic behaviours through reversible plastic deformation by twinning and spontaneous detwinning upon unloading or heating [18] . Based on the predicted reversible twinning–detwinning behaviour of ultra-thin fcc nanowires, a concept of mechanical energy storage was recently suggested [19] . Until now, understanding on the deformation mechanisms of metal nanowires has been led mainly by atomistic simulations. However, the predictions still need to be verified by experiments, as they are shown to vary depending on the atomic potentials used and the initial configuration of the nanowire in terms of shape, size and defects. In situ mechanical testing in a transmission electron microscope (TEM) is a unique complementary tool to MD simulation that can directly visualize the dislocation processes taking place at similar length scales. Moreover, while MD approaches are suited to handling only small crystals at high strain rates (10 7 –10 9 s −1 ), larger nanowires with diameters up to several hundred nanometres can be tested in the TEM at a laboratory strain rate level (10 −3 –10 −1 s −1 ). Nonetheless, most in situ TEM experiments conducted so far have been limited to the tensile deformation of few 10-nm thick nanowires [20] , [21] , which can address only a part of the active deformation modes predicted by MD simulations. In the present study, in situ TEM observations demonstrate that the deformation mode of Au [110] nanowires changes from dislocation slip to deformation twinning as the loading condition is reversed from compression to tension. Furthermore, by performing cyclic compressive-tensile deformation, we show that once a nanowire has been twinned by the initial tensile loading, the subsequent compressive deformation was carried predominantly by detwinning instead of the expected dislocation slip. This twinning–detwinning behaviour is capable of accommodating large plastic strains (>30%) reversibly and repeatedly over many tension–compression cycles. Crystallographic orientation and shape of Au [110] nanowires We used Au [110] nanowires prepared by two different routes. Intensively used are the monolithic Au [110] nanowires grown vertically on a SrTiO 3 (110) substrate by a vapour phase deposition process [22] , [23] . In order to ensure high crystalline quality and low defect density, the nanowires were grown at a low growth rate. The diameter of the tested nanowires ranged from ~80 nm to 350 nm and the aspect ratio (length-to-diameter ratio) was larger than 5. In addition, Au [110] nanowires grown by molecular beam epitaxy (MBE) were also used. These are much longer and thinner than the former wires and used for dedicated tensile testing [4] . The top end of all [110]-oriented Au nanowires was bound by two inclined {111} faces in a wedge shape ( Fig. 1a ). The side faces consist of four large {111} and two small {100} planes. The faceting by these six transverse side faces results in a truncated rhombic cross-section. According to the Wulff construction, the {100} side faces do exist in the cross-section of Au [110] wires even when the largest reported surface energy of {100} is considered [4] , [24] (see Fig. 1d ). The relative area of the {100} side faces in the grown [110] nanowires was observed to vary from nanowire to nanowire, but remained close to that expected by the Wulff construction. Concerning the effects of the cross-sectional shape on the deformation behaviour of ultra-thin fcc [110] nanowires, one is referred to the MD simulations performed with various cross-sectional shapes [14] , [25] . Although the deformation mechanisms of the 〈110〉{111} rhombic nanowires have significance in their own right, we believe that using the thermodynamically stable and high crystalline nanowires with a cross-sectional shape close to the equilibrium is more relevant for the experimental study of deformation mechanisms. TEM observations of the as-grown Au nanowires at various two-beam diffraction conditions confirmed that they are free from dislocations. For example, the TEM dark-field (DF) images in Fig. 1b,c show no structural defects, only the diffraction fringes associated with the thickness variation along the viewing direction. The possible slip systems are shown using the Thompson tetrahedron [26] in Fig. 1e . The slip systems CB and CA on the (d) as well as BD and AD on the (c) plane have a Schmid factor ( m ) of 0.408, whereas all the others are 0. 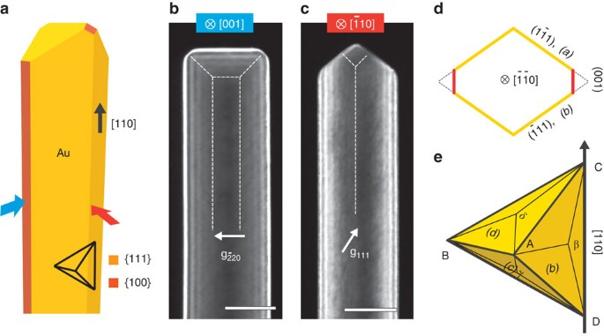Figure 1: Crystallographic orientation, shape and slip systems of the Au [110] nanowires. (a) Schematic illustration of the growth morphology of Au [110] nanowires. The side faces are bound by four large {111} (yellow) and two small {100} faces (red) parallel to the [110] growth direction, resulting in a truncated rhombic cross-sectional shape. The top end of the Au nanowires is bound by two inclined {111} faces in a wedge shape. Small {100} facets are observed to exist where the four {111} facets intersect at the top corners. (b,c) TEM DF images of a pristine Au nanowire recorded using theg=two-beam diffraction condition from the [001] viewing direction, and with theg=111 from thedirection, respectively. Only thickness fringes are visible, without any additional diffraction contrast from dislocations. Scale bars, 100 nm. (d) Equilibrium cross-sectional shape of the Au [110] nanowire calculated by the Wulff construction. (e) Slip systems of the Au [110] nanowires using the Thompson’s tetrahedron. Possible partial dislocations have largely different Schmid factors: Cδ and γD have m =0.471, while δA , δB , Bγ and Aγ have m =0.234 ( Table 1 ). Figure 1: Crystallographic orientation, shape and slip systems of the Au [110] nanowires. ( a ) Schematic illustration of the growth morphology of Au [110] nanowires. The side faces are bound by four large {111} (yellow) and two small {100} faces (red) parallel to the [110] growth direction, resulting in a truncated rhombic cross-sectional shape. The top end of the Au nanowires is bound by two inclined {111} faces in a wedge shape. Small {100} facets are observed to exist where the four {111} facets intersect at the top corners. ( b , c ) TEM DF images of a pristine Au nanowire recorded using the g = two-beam diffraction condition from the [001] viewing direction, and with the g =111 from the direction, respectively. Only thickness fringes are visible, without any additional diffraction contrast from dislocations. Scale bars, 100 nm. ( d ) Equilibrium cross-sectional shape of the Au [110] nanowire calculated by the Wulff construction. ( e ) Slip systems of the Au [110] nanowires using the Thompson’s tetrahedron. Full size image Table 1 Schmid factors of possible slip systems. Full size table Deformation by dislocation slip in compression In our deformation setup the wedge-shaped top end of the nanowire was compressed with a flat diamond punch ( Fig. 2a ), thus the initial deformation was localized near the contact region. Moreover, the strain is highest at the top corner and decreases steeply along the radial and axial directions (one can envision the inverse of a nanoindentation setup). Under such a strong strain gradient condition, the initial compressive deformation began with the emission of small prismatic loops from the top corner (white arrows in Fig. 2b ; Supplementary Movie 1 ). After nucleation, these prismatic loops immediately slipped down the wire to reach a stable position, where they remained stationary until the stress fields of successively generated loops forced them to glide further down. The loops slipped along the wire axis on two parallel sets of ( a ) and ( b ) planes in a jerky manner. 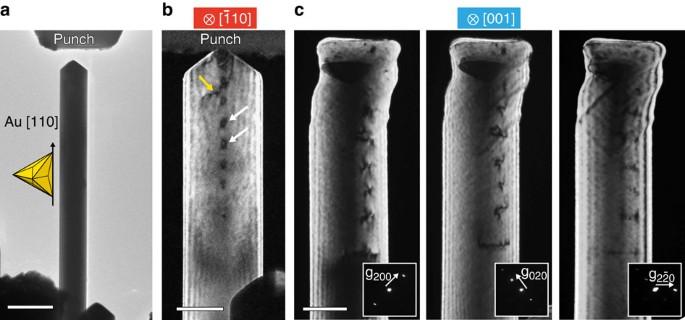Figure 2: Initial plasticity of Au [110] nanowires by prismatic loops. (a) Low-magnification TEM image of the compression setup using a flat diamond punch. Scale bar, 500 nm. (b) TEM DF image showing the initial compressive deformation accommodated by the nucleation of prismatic loops (white arrows) and half-loop shaped dislocations (yellow arrows). Upon emission, these loops slip along the glide planes lying parallel to the loading axis, that is, (a) and (b) planes inFig. 1d. The loops spacing remained in the range of ~50–100 nm, and the dislocation density was measured to be on the order of ~109–1010cm−2. Scale bar, 100 nm. (c) TEM DF images of open prismatic dislocation loops recorded at various two-beam conditions. The dislocations are visible in the first two images recorded atg=200 andg=020. In the last image recorded atg=, the dislocations are invisible. According to theg·binvisibility criterion, the Burgers vector is determined asa/2. The weak residual contrast of the dislocations remained atg=originates from theg·b × ucontrast, refer to Methods for details. Scale bar, 100 nm. Figure 2: Initial plasticity of Au [110] nanowires by prismatic loops. ( a ) Low-magnification TEM image of the compression setup using a flat diamond punch. Scale bar, 500 nm. ( b ) TEM DF image showing the initial compressive deformation accommodated by the nucleation of prismatic loops (white arrows) and half-loop shaped dislocations (yellow arrows). Upon emission, these loops slip along the glide planes lying parallel to the loading axis, that is, ( a ) and ( b ) planes in Fig. 1d . The loops spacing remained in the range of ~50–100 nm, and the dislocation density was measured to be on the order of ~10 9 –10 10 cm −2 . Scale bar, 100 nm. ( c ) TEM DF images of open prismatic dislocation loops recorded at various two-beam conditions. The dislocations are visible in the first two images recorded at g =200 and g =020. In the last image recorded at g = , the dislocations are invisible. According to the g · b invisibility criterion, the Burgers vector is determined as a /2 . The weak residual contrast of the dislocations remained at g = originates from the g · b × u contrast, refer to Methods for details. Scale bar, 100 nm. Full size image Initially, the loops appeared to replicate the circumference of the contact area, but after a certain number of closed loops were punched out (typically <10), there was a clear transition in the nucleation mechanism; open loop dislocations started to bulge out and were then released from the contact area (yellow arrows in Fig. 2b and also in Fig. 3 ). The Burgers vector of these loops was determined to be by applying g · b invisibility criteria to various two-beam DF images ( Fig. 2c ), that is, corresponding to CD in Fig. 1d (refer to the Methods section for a detailed explanation). The Burgers vector of these loops was the same as that of the closed ones. Different from the closed prismatic loops, the free moving ends of the open loops intersected the surface and swept across the top faces before being released, thereby relaxing the strain accumulated beyond the contact area ( Supplementary Movie 1 ). 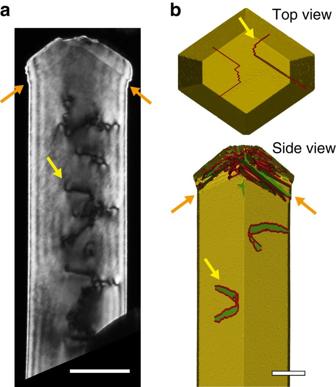Figure 3: Compressive deformation of Au [110] nanowires by dislocation slip processes. (a) TEM DF image showing the emission of half-loop shaped dislocations (yellow arrows) as the contract area broadened. In addition, ordinary dislocation slip occurred through nucleation-glide-escape processes of perfect dislocations, leaving the slip steps along the inclined (c) and (d) planes (orange arrows). Scale bar, 100 nm. (b) MD simulation showing the emission of half-loops (yellow arrow) and ordinary dislocation slip (orange arrows) along the inclined (c) and (d) planes during the initial compression (the flat punch indenter is not shown). The top view image at a perspective angle clearly shows that the moving arms of half-loop shaped dislocations terminate at side surfaces. Scale bar, 20 nm. Figure 3: Compressive deformation of Au [110] nanowires by dislocation slip processes. ( a ) TEM DF image showing the emission of half-loop shaped dislocations (yellow arrows) as the contract area broadened. In addition, ordinary dislocation slip occurred through nucleation-glide-escape processes of perfect dislocations, leaving the slip steps along the inclined ( c ) and ( d ) planes (orange arrows). Scale bar, 100 nm. ( b ) MD simulation showing the emission of half-loops (yellow arrow) and ordinary dislocation slip (orange arrows) along the inclined ( c ) and ( d ) planes during the initial compression (the flat punch indenter is not shown). The top view image at a perspective angle clearly shows that the moving arms of half-loop shaped dislocations terminate at side surfaces. Scale bar, 20 nm. Full size image After the initial deformation by prismatic dislocation loops that had flattened and widened the top end of the nanowire, ordinary dislocation slip became activated along the inclined (c) and (d) planes (orange arrows in Fig. 3a and Supplementary Movie 1 ). In contrast to the prismatic dislocation loops, dislocations on these planes slipped out of the nanowire quickly due to the limited available glide distance (for example, about 170 nm for the nanowire with a diameter of 140 nm shown in Fig. 3a ). This slip process occurred too fast to capture the underlying mechanisms, but the remaining slip steps give an estimate of the total number of dislocations that escaped. To gain further insight into the deformation mechanisms, we performed atomistic simulations on [110]-oriented Au nanowires with a diameter of 50 nm and a length of 200 nm, modelled with the exact geometry and aspect ratio of the experimental nanowires. The simulations reproduced fundamentally the same dislocation processes, namely, the nucleation of perfect dislocations in forms of (open) prismatic dislocation loops ( Fig. 3b ). The simulation also verified that the slip along the (c) and (d) planes occurs by consecutive processes of nucleation-glide-escape of perfect dislocations ( Supplementary Movie 2 ). Slight differences between the MD simulations and the experiments are most probably due to the stiff simulation setup that does not allow for lateral displacements compared with the experiments. The wedge-shaped wire top was deformed to a mushroom-like flat shape as the two localized dislocation processes continued in a complementary manner (for example, Fig. 4a ). As the contact area was extended beyond the cross-section of the nanowire, ordinary dislocation slip (that is, slip along the (c) and (d) planes) dominated the compressive deformation ( Fig. 4a–c and Supplementary Movie 3 ). When this condition was reached, the force-displacement curve exhibited an alternation between elastic loading and load drops, which is a signature of discrete slip bursts ( Fig. 4g ). The observed slip bursts are similar to what was frequently observed during the source-controlled deformation of submicron single crystal pillars [6] , [8] , [27] . It is worth noting that the dislocation density remained as high as ~10 9 –10 10 cm −2 during the compressive deformation due to the previously generated prismatic loops. However, the force-displacement curve indicated that these loops do not seem to lead to strain hardening of the nanowire. Moreover, some of the open prismatic loops assisted the dislocation slip process on the (c) and (d) planes by escaping the nanowire along the corresponding slip planes (see the last scene of Supplementary Movie 1 ). The atomistic details of the underlying dislocation processes are currently unclear and require further elaborate simulation. In addition, arrays of open loops were often introduced asymmetrically in one side of the nanowire to accommodate bending of the nanowire during the elastic loading stages (orange arrows in Fig. 4a ) after slip bursts. 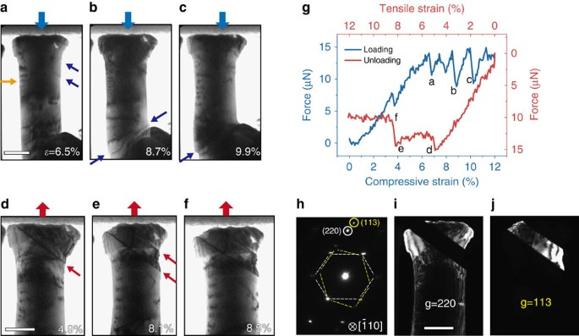Figure 4: Transition of deformation mechanism by load reversal. (a–c) Sequence of TEM images captured right after the load drops occurred at compressive strains ofɛ=6.5%, 8.7% and 9.9%, respectively. Slip steps are indicated by blue arrows. The GNDs that accommodate the bending of nanowire are indicated by orange arrows. Scale bar, 100 nm. (d–f) Sequence of TEM images captured during tensile deformation, showing the nucleation and extension of a nanotwin. The deformation twinning initiated with the formation of a thin twin band (red arrow) and extended to a nanotwin. Scale bar, 100 nm. (g) Force-displacement data obtained during compressive (blue) and subsequent tensile loading (red) (seeSupplementary Movie 3). Note that the zero stress point drifted off from the initial calibration due to electron beam charging effects. (h) Selected area electron diffraction pattern taken at thezone axis showing a Σ3twin relationship. The diffraction spots used for the TEM DF images are marked by circles (the primary reflection by a white circle and the twin reflections by a yellow circle, respectively). (i) TEM DF image formed by using theg=220 primary reflection. Scale bar, 100 nm. (j) TEM DF image formed by using theg=113 twin reflection. Scale bar, 100 nm. Figure 4: Transition of deformation mechanism by load reversal. ( a – c ) Sequence of TEM images captured right after the load drops occurred at compressive strains of ɛ =6.5%, 8.7% and 9.9%, respectively. Slip steps are indicated by blue arrows. The GNDs that accommodate the bending of nanowire are indicated by orange arrows. Scale bar, 100 nm. ( d – f ) Sequence of TEM images captured during tensile deformation, showing the nucleation and extension of a nanotwin. The deformation twinning initiated with the formation of a thin twin band (red arrow) and extended to a nanotwin. Scale bar, 100 nm. ( g ) Force-displacement data obtained during compressive (blue) and subsequent tensile loading (red) (see Supplementary Movie 3 ). Note that the zero stress point drifted off from the initial calibration due to electron beam charging effects. ( h ) Selected area electron diffraction pattern taken at the zone axis showing a Σ3 twin relationship. The diffraction spots used for the TEM DF images are marked by circles (the primary reflection by a white circle and the twin reflections by a yellow circle, respectively). ( i ) TEM DF image formed by using the g =220 primary reflection. Scale bar, 100 nm. ( j ) TEM DF image formed by using the g =113 twin reflection. Scale bar, 100 nm. Full size image Deformation by twinning in tension The adhesive contact formed between nanowire and punch during the compressive deformation allowed tensile loading of the nanowire simply by reversing the loading direction. At the initial stage of tensile deformation, the dislocations existing from the previous compressive loading slipped back. Later, the nanowire deformed predominantly by deformation twinning (see Supplementary Movie 3 ). The deformation twinning started with the formation of a thin twin band on an inclined ( c ) plane near the tensile grip (red arrow in Fig. 4d ). Note that the onset load (or stress) for twinning in this pre-strained (compressed) nanowire was much lower than that required for a pristine Au [110] nanowire [23] , [28] , presumably because the preexisting slip steps on the side faces acted as local stress concentrations. Further straining extended the thin twin band into a nano-scale twin (hereafter referred to as nanotwin) ( Fig. 4e ). Extension of the nanotwin occurred at an even lower load level than that required for the twin initiation ( Fig. 4g ), which agrees well with previous MD simulations [13] , [28] , [29] and experiments [23] , [28] , [30] . The Σ3 twin relationship was confirmed by forming TEM DF images using the primary (220) and the twinned (113) reflections, as shown in Fig. 4h–j . The twinning phenomena of fcc [110] nanowires have been observed predominately through MD simulations of the rhombic wires with {111} side faces [13] , [15] . The truncation by {100} side faces must be an important factor governing the stable growth of twins, since the {100} side faces have to be reoriented to the high-energy {110} surfaces upon twinning [25] . According to the MD simulation reported by Leach et al . [25] , only the nanowires with a certain extent of {100} side faces are able to deform by twinning that results in the transformation of the {111} surfaces to {100} and the {100} surface to {110}. Recent mechanical testing of truncated fcc nanowires with {100} side faces showed deformation twinning in tension [4] , [28] , in accordance with our observations. 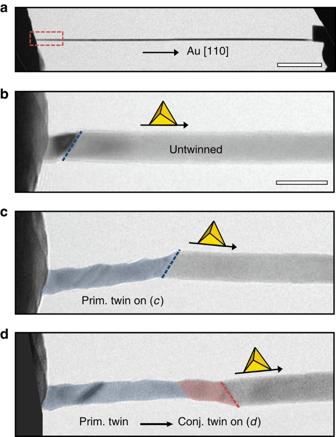Figure 5: Alternate activation of slip systems during twinning of a 20 nm thick Au [110] nanowire. (a) Low-magnification TEM image showing the tensile testing setup for the MBE-grown nanowire that was prepared by utilizing a cold welding method. The tensile deformation was localized near the left tension grip, outlined by dotted red lines. Scale bar, 200 nm. (b–d) Sequence of TEM images captured during the tensile deformation of the Au nanowire by deformation twinning (Supplementary Movie 4). Initial deformation started by the nucleation and growth of a twin along thecplane that is defined as the primary twin (indicated as ‘Prim. twin’ and highlighted in blue). After the primary twin extends over ~60 nm, the twin boundary transits and propagates along the (d) plane, which corresponds to the conjugate twin (indicated as ‘Conj. twin’ and highlighted in red). The bending of the untwinned region ahead of the moving twin boundary causes a strain contrast and is depicted by the corresponding rotation of the Thomson’s tetrahedron. Scale bars, 20 nm. Figure 5 shows the twinning behaviour of a ~20-nm thick nanowire under tension ( Supplementary Movie 4 ). After the extension of a twin along the primary slip system over a certain distance (~60 nm) ( Fig. 5b,c ), the conjugate slip system was activated, stimulated by the internal bending stress ( Fig. 5d ). In the course of tensile deformation, the alternate activation of primary and conjugate twins can effectively relieve the internal bending stress. The bending stress arising in a nanowire upon twinning may vary depending on the applied load, the length and width of the twinned section, the crystal orientation and the lateral compliance of the specimen/grip assembly [28] . Figure 5: Alternate activation of slip systems during twinning of a 20 nm thick Au [110] nanowire. ( a ) Low-magnification TEM image showing the tensile testing setup for the MBE-grown nanowire that was prepared by utilizing a cold welding method. The tensile deformation was localized near the left tension grip, outlined by dotted red lines. Scale bar, 200 nm. ( b – d ) Sequence of TEM images captured during the tensile deformation of the Au nanowire by deformation twinning ( Supplementary Movie 4 ). Initial deformation started by the nucleation and growth of a twin along the c plane that is defined as the primary twin (indicated as ‘Prim. twin’ and highlighted in blue). After the primary twin extends over ~60 nm, the twin boundary transits and propagates along the ( d ) plane, which corresponds to the conjugate twin (indicated as ‘Conj. twin’ and highlighted in red). The bending of the untwinned region ahead of the moving twin boundary causes a strain contrast and is depicted by the corresponding rotation of the Thomson’s tetrahedron. Scale bars, 20 nm. Full size image It is important to consider the persistence of a single-twin variant during twinning, either by continuous extension of a single twin ( Figs 4d–f and 5b–c ), or by the formation of parallel nanotwin lamellae [28] as shown in Fig. 6a , since the crystal reorientation caused by twinning induces nanowire bending ( Fig. 5b,c ); the twinned region is rotated with respect to the untwinned part by an angle corresponding to the change of the [110] axial direction to the direction (~19.5°) [29] . If a nanowire is firmly clamped, it progressively bends across the twin boundary during growth of the twin. The bending alters the Schmid factors of the slip systems in the untwinned region ahead of the twin boundary (usually tending to increase that of the conjugate slip system over the primary one). As the magnitude of internal bending stress increases with increasing twin length, the conjugate twin can be activated ( Supplementary Movie 4 ). 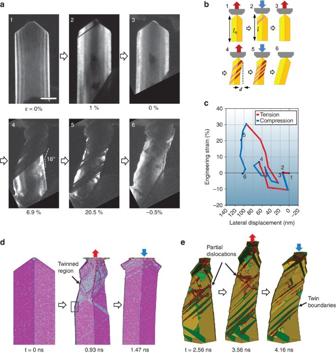Figure 6: Reversible plastic deformation through twinning and detwinning transition. (a) Series of TEM DF images captured from the real-time TEM movie (Supplementary Movie 5) during cyclic tension–compression. Upon the first tensile loading, a single nanotwin was formed near the tensile grip (image 1 to 2) and then erased completely by detwinning during subsequent compression (image 2 to 3). Subsequent tensile deformation was dominated by the successive nucleation and extension of parallel nanotwins along the same slip system (image 4 to 5). As the nanotwins spread over the full gauge length of nanowire while maintaining the same twin variant, the wire axis of the twinned part was rotated by ~18°. A large strain of ~30% was accommodated by twinning and then recovered by detwinning during subsequent compression (image 6). Scale bar, 100 nm. (b) Schematics illustrating the corresponding loading condition for each TEM image in (a). (c) Plot of the axial strain versus the lateral displacement during the cyclic loading. (d) Snapshots from MD simulations showing the tensile deformation by twinning and subsequent detwinning of the twinned nanowire upon compressive loading. The colour coding represents the coordination number; magenta: 9 for the {111} surface atoms; grey: 8 for the {100} surface atoms in the twinned part. (e) Snapshots from MD simulations showing the growth of twins in tension and detwinning in compression by the glide of partial dislocations at the twin boundaries. Dislocations are shown as red lines and the twin boundaries in green. Figure 6: Reversible plastic deformation through twinning and detwinning transition. ( a ) Series of TEM DF images captured from the real-time TEM movie ( Supplementary Movie 5 ) during cyclic tension–compression. Upon the first tensile loading, a single nanotwin was formed near the tensile grip (image 1 to 2) and then erased completely by detwinning during subsequent compression (image 2 to 3). Subsequent tensile deformation was dominated by the successive nucleation and extension of parallel nanotwins along the same slip system (image 4 to 5). As the nanotwins spread over the full gauge length of nanowire while maintaining the same twin variant, the wire axis of the twinned part was rotated by ~18°. A large strain of ~30% was accommodated by twinning and then recovered by detwinning during subsequent compression (image 6). Scale bar, 100 nm. ( b ) Schematics illustrating the corresponding loading condition for each TEM image in ( a ). ( c ) Plot of the axial strain versus the lateral displacement during the cyclic loading. ( d ) Snapshots from MD simulations showing the tensile deformation by twinning and subsequent detwinning of the twinned nanowire upon compressive loading. The colour coding represents the coordination number; magenta: 9 for the {111} surface atoms; grey: 8 for the {100} surface atoms in the twinned part. ( e ) Snapshots from MD simulations showing the growth of twins in tension and detwinning in compression by the glide of partial dislocations at the twin boundaries. Dislocations are shown as red lines and the twin boundaries in green. Full size image Reversible twinning and detwinning under cyclic tensile and compressive loading When a twinned nanowire was subsequently compressed, the twins were observed to shrink progressively from their boundaries and eventually disappeared. In other words, the compressive strain was accommodated by a detwinning process ( Fig. 6a and Supplementary Movie 5 ). This detwinning behaviour is in a stark contrast to the dislocation slip governing the first compressive deformation of the pristine Au nanowire. When the loading direction was subsequently reversed to pull the detwinned nanowire into tension, it deformed again by twinning ( Fig. 6a and Supplementary Movie 5 ). There have been MD simulations reporting the spontaneous detwinning of ultra-thin fcc [110] nanowires driven by the surface stress [18] . However, for all nanowires studied in the present case, the resolved shear stress on the twin boundaries overrides the contribution of surface stress on the side faces by far. In the case of the nanowire shown in Fig. 6a , the twinning occurred by successive nucleation and extension of parallel nanotwins of the same twin variant throughout the length of the nanowire. As a consequence, the twinned region (here referred to the region consisting of multiple nanotwin lamellae) was rotated by ~18° with respect to the untwinned part ( Fig. 6a ), but without causing a significant bending of the nanowire. The persistence of a single-twin variant without bending of the nanowire is closely related to the mechanical boundary conditions of this nanowire. The bottom mount of the nanowire, connected to the piezo stage at the end, is relatively free to slide with respect to the top end. Therefore, it can accommodate the lateral displacement caused by the crystal reorientation of due to twinning. Moreover, the adhesion-based top tension grip of this nanowire in particular allows the rotation of the wire axis from the loading axis by behaving like a pivotal joint. These boundary conditions ensure the successive nucleation and stable growth of nanotwins with the same twin variant and prevent the nanowire from bending. The axial (engineering) strain and the lateral displacement were measured and plotted in Fig. 6c . The axial strain is defined as ( l−l 0 )/ l 0 , where l 0 and l are the wire length before and after deformation. The lateral displacement d caused by the reorientation was measured at the bottom end of the nanowire (see Methods). For this particular specimen and deformation setup, the twinning–detwinning transition was reversible and repeatable over four tension–compression cycles, which did accommodate large strains up to ~30%, while exhibiting a substantial lateral displacement of ~120 nm over the active deformation gauge length of ~750 nm (that is, the full length of the nanowire). The maximum strain attainable by this type of reversible deformation should be comparable with that obtained by the simple reorientation of a rhombic 〈110〉{111} nanowire to a 〈100〉{100} nanowire, which corresponds to 41.4% [15] . Interestingly, the MD simulations on Au whiskers of similar shape and identical orientation showed a failure strain of 59% [28] . Discussion The transition of deformation mechanism upon changing the loading direction is a direct consequence of the interchange in Schmid factor between the leading and trailing partial dislocations. In compression, the Schmid factors for the potential leading (for example, Cδ in Fig. 1d ) and trailing ( δA ) partial dislocations are m =0.234 and 0.471 ( Table 1 ), respectively. Thus, once a leading partial dislocation is nucleated in compression, it is swiftly followed by a trailing partial dislocation, resulting in full dislocation slip (for example, CA ). However, the order of Schmid factors are reversed in tension, that is, m =0.471 and 0.234 for the potential leading ( Aδ ) and trailing ( δC ) partial dislocations, respectively. This indicates that in tension, the successive nucleation of a trailing partial dislocation is not preferred. Instead, the consecutive nucleation of leading partial dislocations is favored, each of which trails a stacking fault behind, satisfying a requirement for forming deformation twins. This emphasizes the importance of the orientation of the loading axis with respect to the slip systems in addition to the material properties (stacking-fault and twin-fault energies) in determining whether dislocation slip or deformation twinning will be the dominant deformation mechanisms. Although the Schmid law is valid for the nanowire sizes studied in this work, it may not be valid below a certain nanowire diameter [13] , [15] . On the contrary, the transition from twinning to dislocation slip might occur for the tensile deformation of thicker [110] nanowires as a result of competition between the reduced stresses required to bow a full dislocation across the nanowire width and the large energy penalty of forming the stacking faults required for the commencement of twinning [9] , [10] . As unambiguously shown in our experiments, once twin boundaries are present in an Au [110] nanowire, the subsequent compressive deformation favored detwinning over dislocation slip. Since twins are already present, there is no need to generate a leading partial dislocation. Instead, a trailing partial dislocation can directly annihilate the stacking fault on the twin boundary ( Fig. 6e ). In other words, if there is a twin boundary, a trailing partial dislocation can be directly nucleated because of the high Schmid factor ( m =0.471 regarding the original wire orientation; Table 1 ) for this process, reducing the width of the twin by one atomic layer. Therefore, the compressive deformation is carried out preferentially at the twin boundary by trailing partial dislocations ( δA ) at a much lower stress level ( Fig. 4g ). The onset of cyclic deformation, either by slip in compression or twinning in tension, requires high stress. Once initiated, however, subsequent cyclic deformation by twinning–detwinning occurs at a relatively lower stress level (see unloading curve in Fig. 4g ). The slip steps formed at the corners of the side surfaces provide preferred nucleation sites for partial dislocations on atomically adjacent planes (see Fig. 7b,d ); they can act as local stress concentrations and also lower the step energy cost in the dislocation nucleation process [31] . Once a two-layer embryonic twin has formed, only the energy to nucleate a partial dislocation is required for the propagation of the twin boundary, not the stacking-fault energy. In the detwinning case, the successive nucleation of partial dislocations on the adjacent planes can collectively reorient the side surfaces from the {100}-dominant configuration back to the original {111}-dominant facets. All these energetic considerations favour the growth and shrinkage of nanotwins over slip by isolated partial dislocations, that is, partial slip. Moreover, considerations based on the twinnability criteria also predict that twinning is favored over partial slip in Au [110] nanowires [15] . As the cyclic deformation continues, the surface becomes rougher with more slip steps, leading to an increase of the twin density and decrease of the twin lamella width ( Fig. 6a and Supplementary Movie 5 ). The MD simulations further support the preferential activation of the twinning and detwinning processes and the reversible transition between the two mechanisms during cyclic tension–compression loading ( Fig. 6d,e ; Supplementary Movie 6 ). 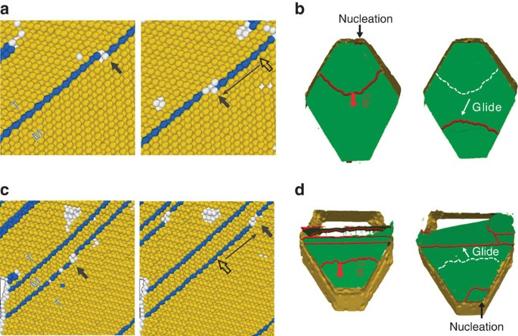Figure 7: Atomic scale mechanisms of twinning and detwinning processes. MD simulation showing the twinning and detwinning processes by the nucleation and glide of partial dislocations. (a,b) Growth of a twin under tension by successive glide of partial dislocations on the adjacent plane. (c,d) Detwinning by reverse glide of partial dislocations with the same Burgers vector as the twinning partial dislocations. Similar to the twinning partial dislocations, the detwinning partial dislocations are nucleated at the intersection of the twin boundary with the surface edges. The dislocations are indicated by black arrows in the side view and highlighted as red lines in the top view. What distinguishes twinning from detwinning is the opposite slip directions each of which has the same Schmid factor ofm=0.471 under the respective loading condition. Colour coding according to the coordination number; yellow: FCC, blue: HCP, white: others. Figure 7a–d present the detailed atomic scale analysis of the dislocation processes that occur at a twin boundary (boxed area of Fig. 6d ) during twinning and detwinning. Under tensile stress, a twinning partial dislocation (corresponding to white coloured atoms) glided downward on the twin boundary, thereby leading to the layer-by-layer growth of the twin ( Fig. 7a ). The detailed analysis [32] of this partial dislocation identifies the Burgers vectors of ( Fig. 7b ). In the detwinning process, as shown in Fig. 7c,d , a partial dislocation glides in the opposite direction. Thus, detwinning is just the opposite of the layer-by-layer twin growth, removing one twin layer after the other by the reverse glide of partial dislocations having the same Burgers vector as the twinning partial dislocations. Figure 7: Atomic scale mechanisms of twinning and detwinning processes. MD simulation showing the twinning and detwinning processes by the nucleation and glide of partial dislocations. ( a , b ) Growth of a twin under tension by successive glide of partial dislocations on the adjacent plane. ( c , d ) Detwinning by reverse glide of partial dislocations with the same Burgers vector as the twinning partial dislocations. Similar to the twinning partial dislocations, the detwinning partial dislocations are nucleated at the intersection of the twin boundary with the surface edges. The dislocations are indicated by black arrows in the side view and highlighted as red lines in the top view. What distinguishes twinning from detwinning is the opposite slip directions each of which has the same Schmid factor of m =0.471 under the respective loading condition. Colour coding according to the coordination number; yellow: FCC, blue: HCP, white: others. Full size image The deformation behaviour of Au nanowires during plastic flow is strongly affected by the boundary conditions of the mechanical testing setup. In the course of uniaxial loading, the plastic deformation of a nanowire is usually not uniform but often localized, giving rise to a strain gradient across the boundary between deformed and undeformed regions. This gradient, if small, is accommodated by elastic bending. However, as it increases with deformation, plastic deformation will eventually accommodate the strain gradient. Full dislocations can be easily nucleated and glide in compression, acting as geometrically necessary dislocations (GNDs) to accommodate the strain gradient, as seen in the initial compressive deformation and also during the elastic loading stages in discrete slip bursts (orange arrow in Fig. 4a ). In the case of tensile loading, as the twins nucleate and extend their length with maintaining a single-twin variant, the internal bending stress increases with the twin length if both ends of the nanowire are fully clamped and no lateral displacement is allowed. This stimulates the activation of the conjugate slip system to relieve the internal bending stress ( Fig. 5 ). However, if the compliance of the boundary conditions allows for lateral displacement, the twin(s) can continue to grow in a stable manner while preserving the primary slip orientation ( Fig. 6 ). This is desired for applications that require reversible cyclic deformation. An ideal boundary condition would be such that one of the tension grips is free to slide and the other one free to rotate, as in Fig. 6 , ensuring that the crystal reorientation can be repeatedly accommodated. In summary, the present in situ TEM results demonstrate the primary role of the crystallographic orientation of fcc metal nanowires in determining the governing deformation mechanisms under uniaxial loading conditions. Because our TEM implementation allows us to see the dislocation processes directly in real time, we found a number of unexpected phenomena. First, we showed that the strain gradient deformation of nanowires occurs by prismatic loops that are analogous to GNDs in bulk deformation. What is unexpected and different from the existing theory of strain gradient hardening is that the size of GNDs in the nanowire is limited by free surfaces, leading to a transition to open loops and escape through the surfaces, certainly contributing to a softening rather than a hardening effect. Second, we showed the importance of bending (another strain gradient) that inevitably arises due to the crystal reorientation associated with twinning. Third, we demonstrate that Au [110] nanowires deform reversibly by a twinning–detwinning mechanism upon load reversal. The multi-cycle tension-compression tests showed that this process is reversible and not limited to idealized situations as studied in atomistic simulations. Importantly, we can, in a unifying approach, explain the newly observed detwinning deformation using analogous arguments employed to describe the twinning process, rather than requiring another specialized theory. In situ TEM The Au [110] nanowires for in situ TEM deformation experiments were prepared by cutting their supporting SrTiO 3 (110) substrate into an ~500-μm thick slice using a low-speed diamond saw. In order to prevent contamination of the Au nanowire surfaces during cutting, no lubricating or cooling agent was used. After dry cutting of the substrate, the Au nanowires were observed to exist stable on the substrate without being damaged or contaminated. The slice was subsequently affixed to a half-circle Cu grid using a silver epoxy. In order to access the cross-sectional view along the [001] and directions of the nanowire in TEM, specimens were prepared along these two separate cross-sectional directions. A nanoindentation TEM holder (Nanofactory) equipped with a diamond flat punch was used for the compression test, which facilitates the simultaneous acquisition of force-displacement curves and real-time TEM movies during deformation. Mechanical testing was carried out by following the prescribed loading–unloading scheme in a displacement-controlled mode to gain a complete set of mechanical data and also by manual control of tip displacements to observe dislocation processes in greater detail. After compression, the adhesion arising between the compressed nanowire tip and the diamond punch allowed tensile deformation of the nanowire during unloading. For the dedicated tensile testing of the long MBE-grown nanowires, a cold welding method was used to fix them to the tension grips [33] . The experiments were carried out in a field emission TEM operated at 200 kV (JEM-2100F, JEOL). Real-time movies were acquired with a charge-coupled device camera (ORIUS 200D, Gatan) at 25 frames per second. Determination of the Burgers vector of prismatic loops In order to identify the Burgers vector of the prismatic dislocations, the g · b invisibility criterion was applied. An array of open prismatic dislocation loops was observed in three different two-beam conditions in DF mode ( Fig. 2c ). The open loop dislocations are visible at g =020 and at g =200. On the other hand, the dislocations are almost invisible at , demonstrating that the Burgers vector is perpendicular to this g vector. In fcc crystals, there are six possible Burgers vectors b for a perfect dislocation. Since only b = a /2 fulfills g · b =0 for and at the same time g · b ≠0 for g =020 and 200, the Burgers vector of the prismatic dislocation loops is determined as b = a /2 , that is opposite to the [110] growth direction of the nanowire. The residual contrast of the loops remaining at condition is due to g · b × u contrast, where u is the line vector of the dislocation. In the case of pure edge dislocations, g · b × u contrast arises even though the two-beam conditions satisfies the g · b =0, since the buckled dislocation glide plane can change the diffraction condition. For a circular shape of dislocation loops as in the present case, there must be some region where b × u is parallel to the g , so that dislocation contrast remains visible. Strain and displacement measurement The cyclic tension–compression deformation (shown in Fig. 6 and Supplementary Movie 5 ) was conducted in manual displacement-controlled mode. The displacement shown in Fig. 6 was measured by using a digital image correlation method. In order to measure the axial strain and the lateral displacement between punch and nanowire, the small Au particle residue remaining on the diamond punch and the slip trace remaining stable on the nanowire surface were used as reference markers. The relative displacement of both features was measured in 29 selected frame images extracted from the real-time movie ( Supplementary Movie 5 ) and their x and y pixel coordinates were processed and converted to the engineering strain and lateral displacement, respectively. Simulation setup and methods MD simulations of Au nanowires were performed using the embedded atom method potential published by Park and Zimmerman [34] . It has been adjusted to reproduce the intrinsic stacking-fault energy and the surface energies. Two wires were modelled following the experimental geometry shown in Fig. 1 . The thin wire has a diameter (measured between {100} facets) of 25 nm and a length of 200 nm. The intersection between the top {111} facets (between planes (d) and (c) in Fig.1d ) was cut to expose a 1.4 nm wide flat (110) surface. The width of the thick wire is 50 nm, whereas the length is 200 nm, maintaining an aspect ratio of about 1:4. The intersection between the top {111} facets (between planes (d) and (c) in Fig. 1 ) was rounded off with a radius of curvature of 3 nm. A flat punch indenter was created by melting a 76 × 76 × 1.4 nm 3 slab of gold atoms and fixing their positions. Similarly, atoms in a layer corresponding two times the cutoff radius of the potential ( r c =0.55 nm) were fixed. The indenter was initially positioned 0.56 nm above the top of the wires. The total simulation setup contains more than 4.4 million atoms for the thin wire and more than 175 million atoms for the thick wire. The entire structures were optimized using FIRE [35] , homogeneously expanded to the lattice constant of the potential at 300 K, and equilibrated for 20 ps at 300 K using standard MD. The temperature in the following MD runs was controlled using the Nosé-Hoover thermostat [36] . During the compression and subsequent retraction, the indenter was displaced as a rigid body with a velocity of 20 m s −1 , corresponding to a strain rate of 10 8 s −1 . The atomic configurations were analysed with respect to their coordination number and also using the dislocation extraction tool DXA [32] . How to cite this article : Lee, S. et al . Reversible cyclic deformation mechanism of Au nanowires by twinning–detwinning transition evidenced from in situ TEM. Nat. Commun. 5:3033 doi: 10.1038/ncomms4033 (2014).